Identification and characterization of a human mitochondrial NAD kinase NAD kinase is the sole NADP + biosynthetic enzyme. Despite the great significance of NADP + , to date no mitochondrial NAD kinase has been identified in human, and the source of human mitochondrial NADP + remains elusive. Here we present evidence demonstrating that a human protein of unknown function, C5orf33, is a human mitochondrial NAD kinase; this protein likely represents the missing source of human mitochondrial NADP + . The C5orf33 protein exhibits NAD kinase activity, utilizing ATP or inorganic polyphosphate, and is localized in the mitochondria of human HEK293A cells. C5orf33 mRNA is more abundant than human cytosolic NAD kinase mRNA in almost all tissues examined. We further show by database searches that some animals and protists carry C5orf33 homologues as their sole NADP + biosynthetic enzyme, whereas plants and fungi possess no C5orf33 homologue. These observations provide insights into eukaryotic NADP + biosynthesis, which has pivotal roles in cells and organelles. NAD + , NADP + and their reduced forms (NADH and NADPH) function as cofactor involved in oxidative–reductive reactions [1] , [2] . NAD + and NADH mainly function in catabolic reactions, whereas NADP + and NADPH are involved in anabolic reactions and defence against oxidative stress [3] . NAD + and NADP + are also known to function as substrates in several reactions [1] , [2] , [4] , [5] , [6] , [7] . NAD kinase (NADK; EC 2.7.1.23) is the sole NADP + -biosynthetic enzyme known to catalyse phosphorylation of NAD + to yield NADP + , using ATP or inorganic polyphosphate (poly(P)) as the phosphoryl donor [1] , and has a vital role in the cell. Poly(P) is a linear polymer of orthophosphate residues linked by energy-rich phosphoanhydride bonds; it has been found in bacteria, fungi and tissues of higher plants and animals, including humans [8] , [9] . Some bacterial and archaeal NADKs utilize both poly(P) and ATP as a phosphoryl donor, although all characterized eukaryotic NADKs use ATP, not poly(P) [10] . Moreover, some bacterial and eukaryotic NADKs also catalyse the phosphorylation of NADH by utilizing ATP to yield NADPH (NADH kinase (NADHK; EC 2.7.1.86) reaction) [10] . NADKs that have higher NADHK activity than NADK activity have also been identified, and in some cases classified as NADHK. So far, only mitochondrial Pos5 of the yeast Saccharomyces cerevisiae and peroxisomal NADK3 of the plant Arabidopsis thaliana have been experimentally defined as NADHK [3] , [11] , [12] , [13] . In the case of yeast, in addition to the gene ( POS5 ) encoding mitochondrial Pos5, S. cerevisiae has other two NADK genes ( UTR1 and YEF1 ) encoding cytosolic Utr1 and Yef1 (refs 3 , 14 , 15 ). The NADK triple mutant ( utr1 yef1 pos5 ) is lethal [11] , [16] , [17] , emphasizing the significance of intracellular NADP(H) biosynthesis. The phenotypes of the POS5 mutant ( pos5 ), which are probably caused by decreased mitochondrial NADPH, indicate that Pos5 is responsible for mitochondrial NADP(H) synthesis and again emphasizes the importance of mitochondrial NADP(H) [3] , [11] , [12] , [17] . Moreover, in addition to the gene ( NADK3 ) encoding peroxisomal NADK3, NADK1 and NADK2 have been identified as NADK genes in A. thaliana [13] , [18] . The products of these genes, NADK1 and NADK2, are localized in the cytosol and chloroplast, respectively [19] . In pea leaf, NADP + enters the plant mitochondria [20] ; thus, the NADP + transporter, which is localized in the inner membrane of mitochondria, is responsible for the supply of plant mitochondrial NADP + . In phylogenetic tree analysis, the plant NADK3 homologues, including A. thaliana NADK3, are distinguishable from NADK homologues, including Pos5 and Utr1 (ref. 21 ). However, the structural features of NADK3 homologues have not been reported. In contrast to yeasts and plants, only a single gene encoding NADK has been found in the human genome; the product of this gene, human NADK, is localized to the cytosol [22] , [23] . No mitochondrial NADK has been found in human. Pollak et al. [23] stated that given the vital role of at least two NADK isoforms in yeast, one would certainly expect more than one mammalian NADK isoform; furthermore, any additional NADK isoforms in mammals should have primary structures substantially different from virtually all previously identified enzymes, at least according to the currently available information [1] . An influx of NAD + through human and mammal mitochondrial membrane has been reported [24] , [25] , but the source of human mitochondrial NADP + has remained elusive despite its great significance. In this study, we identified C5orf33, a human protein of unknown function, as an NADK3 homologue, based on homology search using the primary structure of NADK3 of A. thaliana as a query. The C5orf33 protein is a novel human mitochondrial NADK that is responsible for the missing source of mitochondrial NADP + in human cells. C5orf33 is a candidate human mitochondrial NADK A. thaliana NADK3 homologues are distinguishable from NADK homologues on the phylogenetic tree [21] , although there has been no report of the features of the primary structure of NADK3. To obtain more information, we performed a BLASTP [26] search using the primary structure of NADK3 as a query against all organisms in KEGG (Kyoto Encyclopedia of Genes and Genomes website, http://www.genome.jp/kegg/ ); 1,127 proteins were detected as NADK3 homologues ( E -values, e-179 to 9.9) with E -values less than 10. Human C5orf33 protein was unexpectedly detected as the 134th homologue ( E -value, 9e-06), whereas human NADK was detected as the 833rd homologue ( E -value, 0.25). When BLASTP search was conducted using the primary structure of human NADK as a query, human C5orf33 protein was not included in the detected human NADK homologues (total 1,854 proteins; E -values ranging from 0.0 to 6.1) as reported previously [1] , although the C5orf33 protein contains an NADK motif (Pfam, PF01513 (ref. 27 )) ( Fig. 1a ). NADK3 was detected as the 1,817th homologue ( E -value, 0.49) among human NADK homologues. 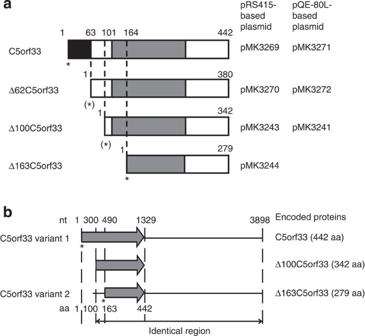Figure 1: Structure of C5orf33 protein. (a) Primary structures of the C5orf33 protein and its truncations. Predicted mitochondrial-targeting sequence and NADK motif are in black and grey, respectively. The amino-acid residue numbers are indicated on the structures. Asterisk in parentheses (*) indicates the start codon found in pMK3270 and pMK3243, but not in the sequence of C5orf33 variant 1. (b) mRNA structures of C5orf33 transcript variants 1 and 2. Grey arrows indicate open reading frames encoding the indicated proteins. The nucleotide (nt) base and amino-acid (aa) residue numbers are shown. The nucleotide sequences indicated by double-headed arrows are identical between variants 1 and 2. The putative start codon (ATG) is denoted by an asterisk (a,b). The nucleotide sequence of C5orf33 variant 2 (62CTTGCATTGAAAGGCTCTAGTTAC85) corresponds to the N-terminal region of the Δ100C5orf33 protein (101LALKGSSY108) (a,b). Figure 1: Structure of C5orf33 protein. ( a ) Primary structures of the C5orf33 protein and its truncations. Predicted mitochondrial-targeting sequence and NADK motif are in black and grey, respectively. The amino-acid residue numbers are indicated on the structures. Asterisk in parentheses (*) indicates the start codon found in pMK3270 and pMK3243, but not in the sequence of C5orf33 variant 1. ( b ) mRNA structures of C5orf33 transcript variants 1 and 2. Grey arrows indicate open reading frames encoding the indicated proteins. The nucleotide (nt) base and amino-acid (aa) residue numbers are shown. The nucleotide sequences indicated by double-headed arrows are identical between variants 1 and 2. The putative start codon (ATG) is denoted by an asterisk ( a , b ). The nucleotide sequence of C5orf33 variant 2 ( 62 CTTGCATTGAAAGGCTCTAGTTAC 85 ) corresponds to the N-terminal region of the Δ100C5orf33 protein ( 101 LALKGSSY 108 ) ( a , b ). Full size image BLASTP analysis showed that the primary structure of human C5orf33 protein (442 amino-acid residues) is 25% identical (37% similar) to that of NADK3 (317 residues). Moreover, using Mitoprot, we identified a mitochondrial-targeting sequence in the N-terminus of the primary structure of the C5orf33 protein [28] ( Fig. 1a ). These features of the primary structure suggested that the C5orf33 protein is a novel candidate human mitochondrial NADK. In vivo assay of NADK activity using S. cerevisiae Two complementary DNAs corresponding to mRNAs from the human C5orf33 gene, transcript variant 1 (accession no. NM_001085411.1) and transcript variant 2 (accession no. NM_153013.3), are deposited in the NCBI database. Transcript variant 1 encodes full-length C5orf33 protein (442 residues) ( Fig. 1a ; Supplementary Fig. S1 ). Transcript variant 2 encodes the C5orf33 protein lacking N-terminal 163 amino acids (Δ163C5orf33 protein, 279 residues) ( Fig. 1a ). Note that variant 2 also is encompassed by Δ100C5orf33 protein (342 residues; Fig. 1a ). The NADK activity of C5orf33, Δ62C5orf33, Δ100C5orf33 and Δ163C5orf33 proteins ( Fig. 1a ) were examined using the S. cerevisiae NADK triple mutant utr1 yef1 pos5 . Δ62C5orf33 protein lacks the 62-residue predicted mitochondrial-targeting sequence. As shown in Fig. 2a , MK1598 cells (an NADK triple mutant having YCplac33- UTR1 ) carrying pRS415 alone were inviable on synthetic complete (SC)+5-fluoroorotic acid (FOA) due to the loss of YCplac33- UTR1 and the lethality of the resultant utr1 yef1 pos5 cell [11] . However, MK1598 cells carrying an additional S. cerevisiae mitochondrial NADHK gene ( POS5 ) on pRS415 (pMK2127) were viable on SC+FOA, although YCplac33- UTR1 was dropped ( Fig. 2a ), indicating that the NADHK activity of Pos5 rescued the lethality of the utr1 yef1 pos5 cells. MK1598 cells carrying the gene encoding either the full-length C5orf33 protein (pMK3269) or the Δ62C5orf33 protein (pMK3270) were viable on SC+FOA medium, but those carrying the Δ100C5orf33 gene (pMK3243) or the Δ163C5orf33 gene (pMK3244) were not, indicating that the C5orf33 and Δ62C5orf33 proteins exhibit NADK or NADHK activity. 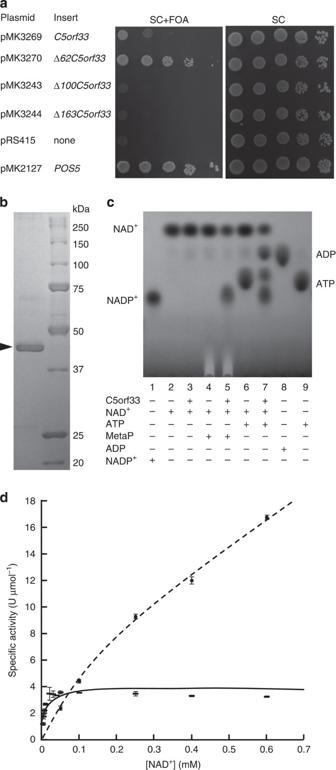Figure 2: NADK activity of C5orf33 protein. (a)In vivoassay of NADK activity of C5orf33 protein.S. cerevisiaeMK1598 cells (an NADK triple mutant having YCplac33-UTR1) carrying the indicated plasmids were spotted onto the solid media and were incubated at 30 °C for 4 days. C5orf33 protein was less effective than Δ62C5orf33 protein in reverting the lethality. We speculate that this is because in the yeast, human C5orf33 is less able to supply cytosolic NADP+than the yeast mitochondrial Pos5 itself. (b) SDS–PAGE of purified C5orf33 protein (arrowhead; 43 kDa). (c) NADK activity of purified C5orf33 protein analysed by TLC in the presence (+) or absence (−) of indicated compounds as described in the Methods. (d) Saturation curves for NAD+of purified human NADK (dashed line)29and C5orf33 protein (line) determined under 8 and 2 mM ATP, respectively. The specific activity (U μmol−1; 1 μmol NADP+produced per 1 min and 1 μmol subunit of the enzyme) was calculated using the subunit molecular mass of C5orf33 protein (45 kDa) or human NADK (43 kDa) (Table 1). Each point represents the average of three determinations; error bars represent s.d. Figure 2: NADK activity of C5orf33 protein. ( a ) In vivo assay of NADK activity of C5orf33 protein. S. cerevisiae MK1598 cells (an NADK triple mutant having YCplac33- UTR1 ) carrying the indicated plasmids were spotted onto the solid media and were incubated at 30 °C for 4 days. C5orf33 protein was less effective than Δ62C5orf33 protein in reverting the lethality. We speculate that this is because in the yeast, human C5orf33 is less able to supply cytosolic NADP + than the yeast mitochondrial Pos5 itself. ( b ) SDS–PAGE of purified C5orf33 protein (arrowhead; 43 kDa). ( c ) NADK activity of purified C5orf33 protein analysed by TLC in the presence (+) or absence (−) of indicated compounds as described in the Methods. ( d ) Saturation curves for NAD + of purified human NADK (dashed line) [29] and C5orf33 protein (line) determined under 8 and 2 mM ATP, respectively. The specific activity (U μmol−1; 1 μmol NADP + produced per 1 min and 1 μmol subunit of the enzyme) was calculated using the subunit molecular mass of C5orf33 protein (45 kDa) or human NADK (43 kDa) ( Table 1 ). Each point represents the average of three determinations; error bars represent s.d. Full size image In vitro NAD(H)K activities of purified C5orf33 To confirm the NADK or NADHK activity of C5orf33 protein in vitro , we expressed recombinant C5orf33 and Δ62C5orf33 proteins in Escherichia coli Rosetta-gami(DE3)pLysS as described in Methods, Supplementary Methods and Supplementary Table S1 . C5orf33 was expressed as an insoluble protein, whereas Δ62C5orf33 protein was partially soluble: ~28% of Δ62C5orf33 protein was soluble and 72% was insoluble ( Supplementary Methods ). We purified the soluble Δ62C5orf33 protein using TALON column chromatography; the resulting product is referred to hereafter as ‘purified C5orf33 protein’ ( Fig. 2b ). SDS–PAGE analysis showed that the molecular mass of the purified C5orf33 protein was 43 kDa, in agreement with the predicted mass (45 kDa; His-tag (1.4 kDa) plus Δ62C5orf33 protein (43.3 kDa)). We assayed the NADK activity of C5orf33 protein using ATP and poly(P) (metaphosphate) as a phosphoryl donor; by thin layer chromatography (TLC) analysis, we detected the formation of NADP + from NAD + and of ADP from ATP ( Fig. 2c ), showing that C5orf33 protein has NADK activity using ATP and poly(P) as phosphoryl donors. The kinetic properties of C5orf33 protein were determined by assay of NADK activity using the continuous method (see Methods), and compared with those of human NADK [29] ( Table 1 ). Both K m (for NAD + ) and V max of C5orf33 protein (0.022±0.001 mM and 0.091±0.001 U mg −1 ) were significantly lower than those of human NADK (1.07 mM and 18.5 U mg −1 ) [29] ( Table 1 ). However, at the physiological concentrations of NAD + found in human mitochondria and cytosol, the NADK activity of C5orf33 protein would be comparable to that of human NADK, as described in the Discussion ( Fig. 2d ). With regard to the substrate specificity of C5orf33 protein, the NADHK activity of C5orf33 protein was only 10% of its NADK activity ( Table 1 ), although the primary structure of C5orf33 protein is similar to that of NADHK (NADK3 (ref. 13 )). ATP-dependent nicotinic acid adenine dinucleotide (NAAD) kinase activity of C5orf33 protein was not detected by TLC. NAAD phosphate (NAADP), the phosphorylated NAAD, is a calcium-mobilizing second messenger in human [6] , [7] . Although NADKs (Utr1 and Yef1) of S. cerevisiae catalyse NAADP synthesis by phosphorylation of NAAD [16] , human NADK has no NAAD phosphorylation activity [22] . Furthermore, TLC analysis detected no phosphorylation of either ADP-ribose, adenosine or 5′-AMP by C5orf33 protein. Sphingosine kinase, diacylglycerol kinase and 6-phosphofructokinase activities of purified C5orf33 protein were assayed by monitoring formation of ADP, as described in Supplementary Methods . Although formation of ADP was observed in the presence of NAD + even in the presence of vehicle alone (16% (v/v) dimethylformamide or 10% (v/v) ethanol), formation of ADP in the presence of sphingosine, diacylglycerol (1,2-dioleoyl- sn -glycerol) and fructose 6-phosphate was not, indicating that purified C5orf33 protein exhibits no sphingosine kinase, diacylglycerol kinase or 6-phosphofructokinase activity, although these kinases have been suggested to be weakly related to NADK with respect to structure and function [30] . Table 1 Properties of C5orf33 protein and human NADK. Full size table On the other hand, as phosphoryl donors, C5orf33 protein could use ATP, other nucleotide triphosphates and poly(P) (metaphosphate, hexametaphosphate and tetrapolyphosphate), but neither ADP, trimetaphosphate, phosphoenolpyruvate nor phosphocreatine ( Table 1 ). It should be noted that C5orf33 protein exhibits a poly(P)-dependent NADK activity comparable to that of its ATP-dependent activity, as it has been postulated that only a subset of bacterial or archaeal NADKs exhibit high poly(P)-dependent NADK activity, whereas eukaryotic NADKs do not [10] . Moreover, C5orf33 protein exhibited a saturation curve with ATP ( Supplementary Fig. S2 ), whereas human NADK exhibited sigmoidal kinetics with ATP [29] . Although human NADK is inhibited by NADH and NADPH, but not NADP + (ref. 29 ), the NADK activity of C5orf33 protein was inhibited by NADH, NADPH and in particular NADP + ( Table 1 ). Mitochondrial localization of C5orf33 protein C5orf33 protein was predicted to be localized in mitochondria because of the presence of a mitochondrial-targeting sequence ( Fig. 1a ). An in vivo assay of C5orf33 protein localization in S. cerevisiae indicated that the C5orf33 protein is localized in mitochondria of S. cerevisiae , whereas Δ62C5orf33 protein that lacks the mitochondrial-targeting sequence is not ( Supplementary Fig. S3 ). To confirm the localization of C5orf33 protein in mitochondria of human cells, HEK293A cells were transiently transfected with a plasmid expressing C terminally FLAG-fused C5orf33 protein or Δ62C5orf33 protein, and observed by fluorescence microscopy after immunostaining ( Fig. 3 ). This observation demonstrated that the C5orf33 protein is localized in mitochondria, whereas Δ62C5orf33 protein is not, confirming that C5orf33 protein is a mitochondrial NADK, and that its N-terminal 62 residues contain a functional mitochondrial-targeting sequence. Moreover, we separated the mitochondrial and cytosolic fractions of siRNA-transfected HEK293A cells and confirmed using anti-C5orf33 antibody that C5orf33 protein was localized in the mitochondrial fraction but not in the cytosolic fraction as below (Fig. 5e). 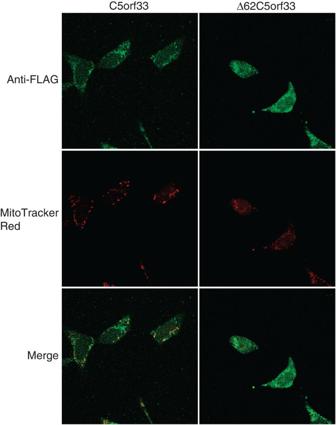Figure 3: Localization of C5orf33 protein in mitochondria of human cells. HEK293A cells were transiently transfected with plasmid expressing C terminally FLAG-tagged C5orf33 or Δ62C5orf33 protein. The cells were fixed and immunostained with a rabbit anti-FLAG primary antibody and AlexaFluor 488-conjugated anti-rabbit secondary antibody. Mitochondria were stained with MitoTracker Red. Figure 3: Localization of C5orf33 protein in mitochondria of human cells. HEK293A cells were transiently transfected with plasmid expressing C terminally FLAG-tagged C5orf33 or Δ62C5orf33 protein. The cells were fixed and immunostained with a rabbit anti-FLAG primary antibody and AlexaFluor 488-conjugated anti-rabbit secondary antibody. Mitochondria were stained with MitoTracker Red. Full size image Widespread expression of C5orf33 mRNA To determine whether C5orf33 gene is transcribed in human tissue under physiological conditions, tissue-specific transcription of mRNAs encoding C5orf33 protein, human NADK and glyceraldehyde 3-phosphate dehydrogenase (GAPDH) were examined by absolute qPCR. The gene encoding GAPDH was selected as a housekeeping gene [31] , [32] . For absolute qPCR, standard curves were created using synthesized mRNAs of the genes encoding C5orf33 proteins, human NADK and GAPDH. As shown in Fig. 4 , the presence of mRNAs encoding C5orf33 protein, human NADK and GAPDH were confirmed in all examined tissues. The relative levels of transcripts of the GAPDH gene in testes, small intestine, colon, stomach and placenta were in agreement with those reported [32] , guaranteeing the quality of the RNAs at least in these tissues. The mRNA levels of C5orf33 protein and human NADK were only a few per cent of the levels of GAPDH (for example, only 2.1% (human NADK gene) and 7.8% ( C5orf33 gene) in brain) ( Fig. 4a ). However, levels of C5orf33 mRNA were higher than those of the human NADK gene in all tissues examined except for colon, spleen and skeletal muscle ( Fig. 4b ). In particular, C5orf33 mRNA levels were significantly higher than human NADK mRNA levels in heart, liver, testes and small intestine. The mRNA levels of both genes were low in skeletal muscle, possibly reflecting the virtual absence of both the pentose phosphate and the fatty acid synthetic pathways in this tissue [22] . 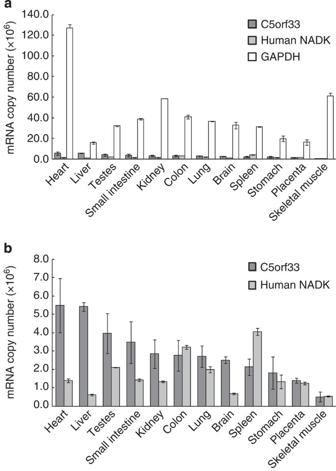Figure 4: Tissue-specific mRNA levels determined by absolute qPCR. mRNAs of C5orf33 protein (dark grey), human NADK (light grey) and GAPDH (white bars) (a); only those of the C5orf33 protein and human NADK are shown in panelb. Means and s.d. of three determinations are shown. Figure 4: Tissue-specific mRNA levels determined by absolute qPCR. mRNAs of C5orf33 protein (dark grey), human NADK (light grey) and GAPDH (white bars) ( a ); only those of the C5orf33 protein and human NADK are shown in panel b . Means and s.d. of three determinations are shown. Full size image C5orf33 affects mitochondrial reactive oxygen species (ROS) generation To obtain information regarding the physiological role of C5orf33 protein, we knocked down the human C5orf33 gene by siRNA transfection of HEK293A cells. Of the six siRNA duplexes we tested ( Supplementary Table S2 ), transfection with siRNA#2 resulted in maximum C5orf33 knockdown (~70% reduction) and siRNA#2 was selected for subsequent knockdown experiments ( Supplementary Methods and Fig. 5a ). 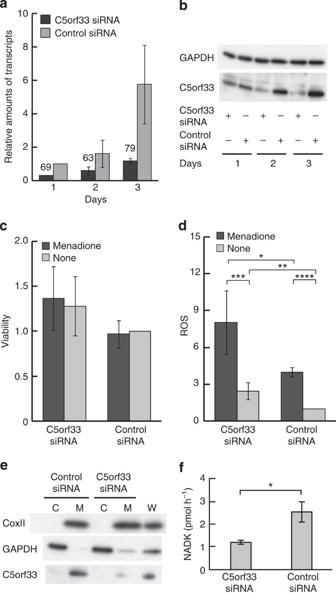Figure 5: siRNA transfection. HEK293A cells were transfected with siRNA#2 against C5orf33 protein (C5orf33 siRNA) or control siRNA, and incubated for 1, 2 and 3 days. (a) Levels of C5orf33 mRNA in the transfected cells are shown as relative values normalized against the level in control siRNA-transfected cells incubated for 1 day after transfection. Knockdowns of 69, 63 and 79% relative to the control, as indicated, were obtained. (b) Expression of C5orf33 protein in the transfected cells. Proteins were analysed by western blotting using anti-C5orf33 and anti-GAPDH antibodies. (c) Viability. Transfected cells incubated for 3 days were treated with 12.5 μM menadione (black bar) or vehicle (0.62% (v/v) dimethyl sulfoxide (DMSO), grey bar) for 20 h, and viability was measured using calcein AM as inSupplementary Methods. Viability was also measured using MTT as inSupplementary Fig. S5. (d) Intracellular ROS levels. Transfected cells incubated for 3 days were incubated with 10 μM 5-(and-6)-chloromethyl-2′,7′-dichlorodihydrofluorescein diacetate, acetyl ester (CM-H2DCFDA) for 30 min, and then treated without (grey bar) or with (black bar) 100 μM menadione for 30 min; intracellular ROS was measured as described inSupplementary Methods.t-test; *P=0.0085, **P=0.0026, ***P=0.0022, ****P=0.0044 × 10−4. Viability and intracellular ROS levels are presented as relative values normalized against their respective levels in control siRNA-transfected cells not treated with menadione; each independent experiment was conducted in duplicate (c,d). (e) Mitochondrial and cytosolic fractions of HEK293A cells that had been incubated for 3 days after transfections. Mitochondrial (M; 1.9 μg) and cytosolic (C; 1.9 μg) fractions and whole cells (W; from 3.3 × 104transfected HEK293A cells) were analysed by western blotting using anti-CoxII, anti-GAPDH and anti-C5orf33 antibodies. CoxII and GAPDH are mitochondrial and cytosolic markers, respectively49. (f) NADK activity of mitochondrial fraction obtained in panele. Mitochondrial NADK activity is expressed as pmol of NADP+formed in 1 h. NADK activity was decreased to 47% upon knockdown of C5orf33.t-test; *P=0.024. Means and s.d. of three independent determinations are shown (a,c,d,f). Figure 5: siRNA transfection. HEK293A cells were transfected with siRNA#2 against C5orf33 protein (C5orf33 siRNA) or control siRNA, and incubated for 1, 2 and 3 days. ( a ) Levels of C5orf33 mRNA in the transfected cells are shown as relative values normalized against the level in control siRNA-transfected cells incubated for 1 day after transfection. Knockdowns of 69, 63 and 79% relative to the control, as indicated, were obtained. ( b ) Expression of C5orf33 protein in the transfected cells. Proteins were analysed by western blotting using anti-C5orf33 and anti-GAPDH antibodies. ( c ) Viability. Transfected cells incubated for 3 days were treated with 12.5 μM menadione (black bar) or vehicle (0.62% (v/v) dimethyl sulfoxide (DMSO), grey bar) for 20 h, and viability was measured using calcein AM as in Supplementary Methods . Viability was also measured using MTT as in Supplementary Fig. S5 . ( d ) Intracellular ROS levels. Transfected cells incubated for 3 days were incubated with 10 μM 5-(and-6)-chloromethyl-2′,7′-dichlorodihydrofluorescein diacetate, acetyl ester (CM-H2DCFDA) for 30 min, and then treated without (grey bar) or with (black bar) 100 μM menadione for 30 min; intracellular ROS was measured as described in Supplementary Methods . t -test; * P =0.0085, ** P =0.0026, *** P =0.0022, **** P =0.0044 × 10 −4 . Viability and intracellular ROS levels are presented as relative values normalized against their respective levels in control siRNA-transfected cells not treated with menadione; each independent experiment was conducted in duplicate ( c , d ). ( e ) Mitochondrial and cytosolic fractions of HEK293A cells that had been incubated for 3 days after transfections. Mitochondrial (M; 1.9 μg) and cytosolic (C; 1.9 μg) fractions and whole cells (W; from 3.3 × 10 4 transfected HEK293A cells) were analysed by western blotting using anti-CoxII, anti-GAPDH and anti-C5orf33 antibodies. CoxII and GAPDH are mitochondrial and cytosolic markers, respectively [49] . ( f ) NADK activity of mitochondrial fraction obtained in panel e . Mitochondrial NADK activity is expressed as pmol of NADP + formed in 1 h. NADK activity was decreased to 47% upon knockdown of C5orf33. t -test; * P =0.024. Means and s.d. of three independent determinations are shown ( a , c , d , f ). Full size image At 2 or 3 days after transfection with siRNA#2, we observed substantial knockdown at the mRNA level ( Fig. 5a ). At 3 days after transfection with either siRNA#2 or MISSION siRNA Universal Negative Control #1 (control siRNA), C5orf33 mRNA levels were higher than those in the corresponding samples that had been incubated for 1 or 2 days after transfection. We also made observations at the protein level, using anti-C5orf33 antibody. We detected obvious knockdown of C5orf33 protein levels at 2 days and especially 3 days after transfection, but not after a 1-day incubation ( Fig. 5b ). In accordance with the relative increase in C5orf33 transcript level 3 days after transfection, the absolute level of C5orf33 protein was highest at this time point. The anti-C5orf33 antibody was specific for purified C5orf33 protein, and did not detect purified human NADK, guaranteeing that the signal we detected accurately represented C5orf33 protein rather than a cross-reaction with NADK ( Supplementary Fig. S4 ). By contrast, the anti-human NADK antibody was nonspecific, detecting both C5orf33 protein and human NADK ( Supplementary Fig. S4 ). Next, we evaluated the effect of the C5orf33 knockdown. Mitochondrial morphology was not affected by knockdown of C5orf33 for 3 days after transfection ( Supplementary Fig. S5 ). During this period, cell viability was also unaffected by knockdown, even in the presence of menadione ( Supplementary Fig. S5 , Fig. 5c ). However, intracellular ROS levels were obviously increased 3 days after knockdown of C5orf33, but not 1 and 2 days, either in the absence or presence of menadione, although ROS levels were higher following menadione treatment ( Supplementary Fig. S5 , Fig. 5d ). Menadione is cytotoxic to various cell lines, including HEK293 (refs 33 , 34 ), and induces apoptosis of cultured cells via elevation of peroxide and superoxide radical levels [35] . Moreover, we separated the mitochondrial and cytosolic fractions of HEK293A cells that had been incubated for 3 days after transfections with siRNA#2 and control siRNA, and again confirmed the mitochondrial localization of C5orf33 protein as well as the knockdown of C5orf33 protein level in mitochondrial fraction of siRNA#2-transfected cells, using anti-C5orf33 antibody ( Fig. 5e ). NADK activity of the mitochondrial fraction was decreased to 47% upon knockdown of C5orf33 ( Fig. 5f ). These observations indicate that C5orf33 protein, that is, human mitochondrial NADK is involved in the regulation of the generation of mitochondrial ROS. Only a single gene encoding NADK has been previously reported to exist in the human genome; the product of this gene, human NADK, is localized in cytosol [22] , [23] . Until now, no mitochondrial NADK had been identified in human. Thus, the source of human mitochondrial NADP(H) has been elusive despite its great significance. In this study, it was revealed that the C5orf33 protein is a novel human mitochondrial NADK that is responsible for the missing source of mitochondrial NADP + in human cells. In HEK293 human cells, the concentration of NAD + in whole cells and mitochondria are 0.37 and 0.25 mM, respectively [36] . Given that mitochondria occupy 15% of the volume of a neuron [37] , we estimated the cytosolic concentration of NAD + to be 0.39 mM. On the other hand, the concentration of ATP, which complexed with magnesium, is estimated to be 2 and 8 mM in mitochondria and cytosol of HeLa cell, respectively [38] . From a saturation curve determined in the presence of 2 mM ATP (the physiological concentration within mitochondria) [38] , we estimated the NADK activity of C5orf33 protein at 0.25 mM NAD + to be 3.5 U per 1 μmol of C5orf33 protein ( Fig. 2d ). In the same manner, the activity of human NADK at 0.39 mM NAD + was estimated to be 12 U per 1 μmol of human NADK subunit in the presence of 8 mM ATP (cytosolic concentration of ATP) [38] ( Fig. 2d ). Moreover, C5orf33 mRNA levels were higher than those of human NADK in almost all tissues ( Fig. 4 ). Collectively, although the V max of C5orf33 protein is significantly lower than that of human NADK ( Table 1 ), under physiological conditions the NADK activity of the C5orf33 protein would be comparable to that of human NADK. BLASTP analyses using each of the primary structures of human C5orf33 protein and human NADK as a query in eukaryotic protein databases detected 107 C5orf33 homologues and 316 human NADK homologues, all of which contain the NADK motif. Phylogenetic trees constructed based on the structures of the 107 proteins as described in Supplementary Methods gave three clades: (i) animal and protist proteins including the human C5orf33 protein (total 65 proteins; E -values from 0.0 to 0.074); (ii) plant proteins including NADK3 (18 proteins; E -values from 8e−11 to 0.049); and (iii) other proteins from several eukaryotes (24 proteins; E -values from 0.017 to 5.4) ( Supplementary Fig. S6 ). These clades were, respectively, designated as (i) C5orf33 homologues, (ii) plant NADK3 homologues and (iii) NADK homologues. The 24 other proteins from several eukaryotes were found in 316 human NADK homologues, gave much lower E -values ranging from 0.0 to 4e−51, and hence were designated as NADK homologues. Predicted mitochondrial-targeting sequences were detected in the primary structures of 38 of 65 C5orf33 homologues, and 4 of 18 plant NADK3 homologues, but not in 24 NADK homologues ( Supplementary Fig. S6 ). Given that eukaryotes consist of animals (for example, vertebrates and insects), protists, plants and fungi, we concluded that animals and protists, but not plants and fungi, have C5orf33 homologues. C5orf33 homologues were found in almost all animals and many protists; 48 of 52 animals and 13 of 29 protists. Although 42 of 52 animals and 5 of 29 protists possess both C5orf33 and NADK homologues, some carry only either a C5orf33 homologue or NADK homologue; one protist ( Naegleria gruberi ) has none ( Supplementary Table S3 ). It is noteworthy that six animals (for example, pig and horse) and eight protists (for example, those in genus Plasmodium ) possess the C5orf33 homologue as sole NADP + biosynthetic enzyme. We performed multiple alignment of the primary structures of human C5orf33 protein, plant NADK3 and nine NADKs ( Supplementary Fig. S7 ). The GGDG motif [39] , NE/D short motif [40] , and the Asp, Thr and Tyr residues (corresponding to Asp-189, Thr-200 and Tyr-202 of Ppnk (NADK of Mycobacterium tuberculosis ) and taking part in the creation of NAD + -binding site) in the NADK-conserved region [40] , [41] are completely conserved in the primary structures of the nine NADKs. In the structure of the C5orf33 protein, although the GGDG motif and NE/D short motif were completely conserved, the Asp, Thr and Tyr residues were not, corresponding instead to Ser-306, Lys-317 and Trp-319. We also found an additional region, termed the C5orf33 additional region, in the structure of the C5orf33 protein. In the sequence of NADK3, the GGDG motif and NE/D short motif are conserved; the Asp, Thr and Tyr residues were Ser-209, Thr-220 and Ala-222; and the NADK3 additional region, which does not correspond to the C5orf33 additional region, is found. In the aligned structures of 65 C5orf33 homologues, the GGDG motif was conserved in 58 of 65 structures; the NE/D short motif was completely conserved (that is, in 65 of 65 structures) ( Supplementary Fig. S7 ). With regard to the Ser-306, Lys-317 and Trp-319 of the human C5orf33 protein, the Ser-306 was conserved as Ser/Thr, the Trp-319 was completely as Trp, although the Lys-317 was not conserved and corresponded to Lys/Ser/Thr/Arg. In the aligned structures of C5orf33 homologues, we found two conserved sequences, motif 1 and motif 2. Motif 1 is PX-GXN(T/S)DP; motif 2 is S-G-X(C/M), where X and hyphen (-) mean hydrophobic (Ile, Phe, Val, Leu and Met) and any amino-acid residues, respectively. Of the aligned 65 sequences, 50 possessed both motifs; of the remaining 15 sequences, 3 contained motif 1 alone, 8 contained motif 2 alone and 4 contained neither. The sequences corresponding to the C5orf33 additional region were also found in 62 of the 65 aligned sequences. In the aligned structures of 18 plant NADK3 homologues, the GGDG motif, the NE/D short motif and motif 1 were completely conserved (in 18 of 18 sequences); motif 2 was almost completely conserved (in 17 of 18 sequences). The Ser-209, Thr-220 and Ala-222 residues of NADK3, corresponding to Asp-189, Thr-200 and Tyr-202 of Ppnk, were conserved as Ser, Thr/Ser and Ala residues. Sequences corresponding to the NADK3 additional region were found in 17 of the 18 sequences ( Supplementary Fig. S7 ). Taken together, these structural features may contribute to the unique properties of human C5orf33 protein, that is, high capacity to utilize poly(P), as well as low K m and low V max , and inhibition by NADP + and of plant NADK3, that is, low K m and high V max for NADH [13] , possibly by using a different set of active-site side chains. Plasmids The plasmids and primers used in this study are listed in Supplementary Tables S4 and S5 . Briefly, pMK2127 is pRS415 carrying the POS5 promoter (P pos5 ) driving POS5 (ref. 11 ). Genes encoding C5orf33 (full-length) and its truncations ( Fig. 1a ) were inserted into downstream P pos5 by replacing POS5 of pMK2127 with these genes. Genes encoding C5orf33 and its deleted proteins were also inserted into BamH I/ Sma I site of pQE-80L (Qiagen), yielding pMK3271, pMK3272 and pMK3241, respectively. These proteins were expressed as His (MRGSHHHHHHGS; 1.4 kDa)-tagged proteins to their N-termini. For expression of C terminally FLAG-tagged human C5orf33 and Δ62C5orf33 proteins in HEK293A cells, cDNAs of human C5orf33 and Δ62C5orf33 were inserted into pFLAG-CMV-5a (Sigma), yielding pMK3602 and pMK3603, respectively. For absolute qPCR, DNA sequences corresponding to cDNA of human GAPDH (1,310 bp; 1,008 bp of GAPDH gene, 5′-flanking 102 bp and 3′-flanking 200 bp), human NADK (3,032 bp; 1,341 bp of human NADK gene, 5′- 42 bp, 3′- 1,649 bp), and C5orf33 variant 1 (3,852 bp; 1,324 bp of C5orf33 gene and 3′- 2,528 bp) were inserted into pBluescript II SK (+), yielding pMK3420, pMK3421 and pMK3422, respectively. Accurate synthesis of all the constructed plasmids was confirmed by DNA sequencing. Yeast strains and cultivations For the cultivation of yeast, standard yeast media (yeast extract/peptone/dextrose, SC and synthetic dextrose media) were used [42] . If required, amino acids were added to synthetic dextrose medium. Liquid medium were solidified using 2% agar. Yeast cells were cultured aerobically at 30 °C. For plasmid shuffling, solid SC medium containing 0.1% FOA (SC+FOA medium) was used. FOA is toxic for the cells containing URA3 (ref. 43 ). S. cerevisiae strains in BY4742 background ( MAT α leu2 Δ 0 lys2 Δ 0 ura3 Δ 0 his3 Δ 1 ) were used. S. cerevisiae MK1598 cell is an NADK triple mutant carrying YCplac33- UTR 1 (BY4742 utr1 Δ:: kanMX4 yef1 Δ:: HIS3 pos5 Δ:: hphMX4 YCplac33- UTR1 ) and is lethal on SC+FOA medium [11] , [16] . In vitro assays NADK activity of purified C5orf33 protein was assayed at 37 °C by the modified continuous method as described previously [29] . Briefly, NADPH formation was continuously measured at A 340 in a reaction mixture (1 ml) containing 5 mM NAD + , 5 mM ATP, 5 mM glucose 6-phosphate, 0.5 U glucose 6-phosphate dehydrogenase (Sigma, St Louis, MD), 5 mM MgCl 2 (40 mM MgCl 2 in the case of the determination of K m and V max for ATP, 20 mM MgCl 2 in that of K m and V max for NAD + ), 100 mM Tris-HCl (pH 8.0) and appropriate concentration of purified protein. NADK activity was also assayed by a stop method as described previously [29] . When NADK activity was analysed by TLC, 5 μl of the reaction mixture containing 5 mM NAD + , 5 mM MgCl 2 , 100 mM Tris–HCl (pH 8.0), 4.8 μg of purified C5orf33 protein and 5 mM ATP or 2.4 mg ml −1 metaphosphate was incubated overnight at 37 °C. Metaphosphate was used at 2.4 mg ml −1 , as 2.4 mg ml −1 sodium tetrapolyphosphate is 5 mM. Authentic compounds and the incubated reaction mixture were spotted onto a TLC glass plate silica gel 60F254 (Merck), dried, developed with a solvent system of isobutyrate—500 mM NH 4 OH (5:3 v/v) [44] and detected by exposure to UV light at 254 nm. The inhibitory effects of NADP + , NADH and NADPH on NADK assay were investigated by a stop method as described previously [29] . The NADHK activity was assayed as described previously [29] in a reaction mixture (1 ml) containing 2 mM NADH, 5 mM ATP, 5 mM MgCl 2 , 100 mM Tris–HCl (pH 8.0) and purified protein. NADK activity of C5orf33 protein was determined by a stop method to compare it with the NADHK activity of the enzyme. NADK activity of mitochondrial fraction was also assayed by the stop method in the reaction mixture as above (40 μl; 5 mM NAD + , 5 mM ATP, 5 mM MgCl 2 , 100 mM Tris–HCl (pH 8.0) and mitochondrial preparations (1.4–35 μg protein)) followed by cycling assay of NADP + as described [45] . In each experiment, the assays were linear with respect to both times (0, 1 and 2 h) and concentrations of mitochondrial preparations (at least two points). One unit of enzyme activity was defined as 1 μmol NADP + or NADPH produced in 1 min at 37 °C; specific activity was expressed in U mg −1 protein, unless otherwise stated. Kinetic values were calculated by fitting the data to the appropriate Michaelis–Menten equations using KaleidaGraph software (Synergy Software). Expression and purification of C5orf33 protein To express C5orf33 and Δ62C5orf33 proteins, MK3274 and MK3275 cells ( E. coli Rosetta-gami(DE3)pLysS (Novagen) cells carrying pMK3271 and pMK3272, respectively) were precultured overnight in 700 ml LB medium (350 ml per 500 ml Sakaguchi flask) supplemented with 100 μg ml −1 ampicillin and 34 μg ml −1 chloramphenicol. The cells collected from the cultures (~75 or 700 ml culture) were inoculated in 1.5 or 13.5 l LB medium (1.5 per 2 l Sakaguchi flask) supplemented with the same antibiotics, and aerobically cultured at 37 °C, until A 600 reached 0.50–1.0. Isopropyl-β- D -thiogalactopyranoside was then added to obtain a final concentration of 25 μM and cell cultivation was continued further at 16 °C under aerobic conditions for 5 days. The conditions for expression were determined as described in Supplementary Methods and Supplementary Table S1 . The crude extract was prepared as described [29] . The Δ62C5orf33 protein was purified as described in Supplementary Methods and the purified protein was regarded as purified C5orf33 protein. Transfection and indirect immunofluorescence microscopy HEK293A cells cultivated in Dulbecco’s modification of Eagle’s minimal essential medium containing 10% fetal bovine serum (DMEMS) supplemented with penicillin (50 μg ml −1 ) and streptomycin (50 μg ml −1 ) on coverslips at 37 °C were transfected with pMK3602 or pMK3603 by Lipofectamine 2000 (Invitrogen), and further cultivated for 2 days at 37 °C. The transfected HEK293A cells were stained with MitoTracker Red CMXRos (500 nM in fresh DMEMS; Molecular Probes) for 45 min, washed with PBS, fixed with 3.7% formaldehyde in PBS, permeabilized with 0.2% Triton X-100 in PBS and blocked using PBS containing 3% bovine serum albumin (BSA). The primary antibody was rabbit anti-FLAG (Sigma) and the secondary antibody was AlexaFluor 488-conjugated anti-rabbit IgG (Invitrogen). Images were acquired using an inverted FV1000-D IX81 (Olympus, Tokyo, Japan) microscope. Absolute qPCR Human total RNAs were purchased from Clontech and Agilent Technologies. The synthesized mRNAs of GAPDH, human NADK, and C5orf33 variant 1 ( Supplementary Fig. S1 ) were prepared using the in vitro Transcription T7 kit (Takara, Otsu, Japan) using as templates, respectively, pMK3420, pMK3421, and pMK3422 linearized by Xho I. The molar concentration of the synthesized mRNAs was calculated from A 260 , and the calculated molecular mass of the synthesized mRNAs (GAPDH, 413 kDa; human NADK, 943 kDa; C5orf33 variant 1, 1,193 kDa). RNA was isolated from siRNA-transfected HEK293A cells using Sepasol-RNA I Super G (Nacalai Tesque, Kyoto, Japan). cDNAs were prepared from RNA and quantitated by absolute qPCR using LineGene (BioFlux, Tokyo, Japan) and SYBR Green Real-time PCR Master Mix (Toyobo) as described in Supplementary Methods . siRNA transfection The siRNA duplexes (Sigma) for knockdown of C5orf33 gene are listed in Supplementary Table S2 . MISSION siRNA Universal Negative Control #1 (control siRNA; Sigma) was used as siRNA duplex for a negative control. Other details were described in Supplementary Methods . Cell viability of the transfected HEK293A cells was measured using 3-(4,5-di-methylthiazol-2-yl)-2,5-diphenyltetrazolium bromide (MTT) or calcein AM (Molecular Probes) and intracellular ROS of the cells were detected as described [23] , [33] , [46] and in Supplementary Methods . Western blotting Proteins were separated by SDS–PAGE [47] and analysed using anti-C5orf33 (Abnova, rabbit polyclonal, 1:2,500 dilution or 1:312,500 as in Supplementary Fig. S4 ), anti-cytochrome C oxidase subunit II (EPR3314) (CoxII; Abcam, rabbit monoclonal, 1:10,000), anti-GAPDH (6C5) (loading control; Abcam, mouse monoclonal, 1:500), anti-human NADK (Abnova, mouse monoclonal, 1:500 as in Supplementary Fig. S4 ) antibodies, which were diluted in Can Get Signal solution 1 (Toyobo). Horseradish peroxide–conjugated anti-rabbit IgG (HRP–anti-rabbit IgG; Amersham Biosciences) and HRP–anti-mouse IgG (Amersham Biosciences) were diluted in Can Get Signal solution 2 (Toyobo) at dilutions of 1:2,000 and 1:10,000, respectively. MagicMark XP Western Standard (Invitrogen) or Precision Plus Protein Standard (Bio-Rad) was used as the standard. For proteins in lysates of transfected HEK293A cells, cells in 4 × 0.6 ml transfection-mixture were collected by treatment with trypsin/EDTA solution (Nacalai Tesque), suspended and boiled for 10 min in 48 μl 1 × SDS buffer. Signal intensities were estimated using ImageQuant TL. Preparation of mitochondria From transfected HEK293A cells, we prepared mitochondria using the Mitochondria Isolation Kit for Cultured Cells (MitoSciences). Details are described in Supplementary Methods . Other analytical methods Protein concentration of the crude extract was determined by the Bradford method [48] , and BSA was used for a standard. The concentration of purified C5orf33 protein was determined using A 280 . A solution containing purified C5orf33 protein with A 280 of 1.0 was calculated to contain 0.9 mg ml −1 from the molar extinction coefficient (51,255), and the calculated molecular mass (46,353 Da) of the C5orf33 protein using ExPASy ( http://br.expasy.org/tools/protparam.html ). The molecular mass of the enzyme was estimated by gel filtration chromatography as described previously [29] . The phylogenetic tree was constructed as described in Supplementary Methods . How to cite this article: Ohashi, K. et al. Identification and characterization of a human mitochondrial NAD kinase. Nat. Commun. 3:1248 doi: 10.1038/ncomms2262 (2012).